Revealing the role of crystal orientation of protective layers for stable zinc anode Rechargeable aqueous zinc-ion batteries are a promising candidate for next-generation energy storage devices. However, their practical application is limited by the severe safety issue caused by uncontrollable dendrite growth on zinc anodes. Here we develop faceted titanium dioxide with relatively low zinc affinity, which can restrict dendrite formation and homogenize zinc deposition when served as the protective layer on zinc anodes. The as-prepared zinc anodes can be stripped and plated steadily for more than 460 h with low voltage hysteresis and flat voltage plateau in symmetric cells. This work reveals the key role of crystal orientation in zinc affinity and its internal mechanism is suitable for various crystal materials applied in the surface modification of other metal anodes such as lithium and sodium. Achieving higher energy density is the main development tendency for the next-generation battery system [1] . Metal anodes, such as lithium (Li), sodium (Na), and zinc (Zn), with high theoretical capacity and low electrochemical potential are considered as the most promising materials to meet this requirement [2] , [3] . However, the electrochemical performance of metal anodes is seriously affected by the dendrite formation during repeated charging and discharging. Metal dendrites are easily detached from anode mainbody and the newly exposed metal would react with electrolyte, leading to low Coulombic efficiency [4] , [5] . More seriously, separators may be punctured by the continuous dendrite growth, which directly causes the short circuit and poor cycle life of batteries [6] , [7] . Therefore, it is important to solve this issue for the industrialization of metal anodes. Many approaches have been developed to achieve safer metal anodes, which mainly focus on two aspects: (1) improving metal deposition on current collectors. Nucleation can be facilitated by a three-dimensional structure with a uniform local electric field [8] , [9] . Some metal-affinity modification layers induced on current collectors are conducive to the adsorption of metal ions, which can guide the deposition and further alleviate dendrites [10] , [11] , [12] . (2) Optimizing the interface between metal and electrolyte. An artificial solid electrolyte interface (SEI) or an additional layer with inferior metal affinity can be applied as a protective layer to restrict dendrite growth [13] , [14] . Metal affinity is a key criterion to judge the applicable functions (guiding or restricting). However, taking titanium dioxide (TiO 2 ) for example, it can be used both for modification of current collectors and protection of metal anodes according to previous reports [15] , [16] , [17] . These results seem contradictory because good metal affinity is required when TiO 2 is used as a decoration on current collectors to homogenize metal deposition while low metal affinity is necessary if it is served as a protective layer [18] , [19] . TiO 2 can be simultaneously applied to two different metal modification strategies with opposite requirements, indicating that there is an ambiguous internal mechanism affecting its metal affinity. Considering that exposed facets of a crystal have a great influence on catalytic activity, metal affinity may be also controllable by adjusting surface exposure [20] , [21] . In this work, the interactions between Zn and different facets of TiO 2 are first investigated by density functional theory (DFT) calculation and it is concluded that the (0 0 1) and (1 0 1) facets of TiO 2 show relatively low Zn affinity. Accordingly, TiO 2 with highly exposed (0 0 1) facet is prepared and applied as the protective layer for Zn metal anodes. The (0 0 1) faceted TiO 2 layer can effectively prevent Zn dendrites from growing vertically and stabilize the interface between anode and electrolyte. As a result, the modified Zn anode exhibits long-term cycle life during Zn stripping and plating. Theoretical analysis and characterization of faceted TiO 2 The mechanism for the interaction between Zn and different facets of TiO 2 is first investigated by DFT calculation. As shown in Fig. 1a–c and Supplementary Figs. 1 and 2 , the models of Zn atoms attached to TiO 2 surfaces and Zn surfaces were constructed. The Zn affinity of TiO 2 surfaces can be judged by comparing the binding energy of Zn atom attached to the TiO 2 surface and Zn surface. It can be considered that a TiO 2 facet is with high Zn affinity if the binding energy of Zn atom attached to the corresponding TiO 2 facet is higher than that on the Zn surface. As summarized in Fig. 1d , the binding energy between Zn atom and TiO 2 (1 0 0) facet is −0.95 eV, higher than that between Zn atom and Zn surfaces (−0.68 and −0.86 eV), indicating that Zn prefers to deposit on TiO 2 (1 0 0) facet in comparison to Zn surface. It is detrimental for a protective layer since this priority can lead to the growth of Zn dendrites upon the layer and deactivate the protective effect. In contrast, there is a weaker absorption of Zn on TiO 2 (0 0 1) and (1 0 1) facets with the binding energy of −0.63 and −0.45 eV, respectively, which is mainly because the more exposure of the lower coordinated Ti on these facets exhibits more intense repulsion to Zn atom [22] . The interaction between Zn and different TiO 2 facets is illustrated in Fig. 1e . According to the above analysis, the facet orientation plays a key role in Zn affinity and suitable materials for a protective layer can be achieved by controlling the exposure of specific facet. Fig. 1: Theoretical simulation and characterization of F-TiO 2 . Calculations models of Zn absorbed on a TiO 2 (0 0 1) facet, b TiO 2 (1 0 0) facet, and c Zn (0 0 1) facet. d Calculated binding energies of Zn atom with different facets. e Schematic illustration of the interaction between Zn and anatase TiO 2 with different exposed facets. f XRD patterns of F-TiO 2 and C-TiO 2 . g – j HRTEM images of F-TiO 2 . Scale bars: 5 nm. Full size image As shown in Fig. 1f , the X-ray diffraction (XRD) patterns of the as-prepared faceted TiO 2 (F-TiO 2 ) and commercial TiO 2 (C-TiO 2 ) can be indexed to anatase TiO 2 . The average thickness along the growth direction of a crystal ( D ) can be calculated by Scherrer equation [23] , [24] : 
    D = Kλ/βcosθ
 (1) where K , λ , β , and θ represent Scherrer constant, the wavelength of X-ray, full width at half maximum (FWHM) of diffraction peak and Bragg angle, respectively. For a specific crystal orientation, the larger FWHM in the XRD pattern indicates the smaller D in this direction, in other words, the larger exposed area of the corresponding facet (Supplementary Fig. 3 ) [25] . Accordingly, the broader (0 0 4) peak in F-TiO 2 demonstrates the larger exposure of (0 0 1) facet and the narrower (2 0 0) peak F-TiO 2 corresponds to the larger crystal size parallel to (0 0 1) facet, which is also the evidence of the relatively higher exposed area of (0 0 1) facet in comparison with C-TiO 2 [26] . In Raman spectra (Supplementary Fig. 4 ), the characteristic peaks of anatase TiO 2 appear at 392.3 cm −1 (symmetric bending vibration, B 1g ), 513.7 cm −1 (antisymmetric bending vibration, A 1g ), 636.5 cm −1 (symmetric stretching vibration, E g ) [27] . The 3-coordinated titanium (Ti) atoms on the (0 0 1) surface (Supplementary Fig. 5a ) with lower coordination number than the 5-coordinated Ti atoms on (1 0 0) surface (Supplementary Fig. 5b ) tend to show stronger bending vibration [28] . Therefore, the weaker A 1g and B 1g peaks in the Raman spectrum of F-TiO 2 suggest its higher exposure of (0 0 1) facet. Transmission electron microscopy (TEM) images (Supplementary Fig. 6 ) clearly show the nanosheet structure of F-TiO 2 with average width and thickness of 50 and 5 nm, respectively. From the side view of F-TiO 2 nanosheet (Fig. 1g ), lattice fringes with a lattice spacing of 0.235 nm are observed, which demonstrates that the [0 0 1] direction is perpendicular to the top surface. Figure 2h is the top-view high-resolution transmission electron microscopy (HRTEM) image of F-TiO 2 nanosheet. 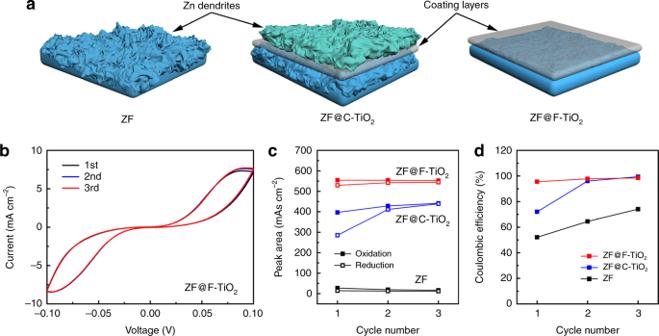Fig. 2: Zn deposition behavior of the prepared anodes. aSchematic illustration of the Zn plating process with different coating layers.bCV curves of Zn–Zn symmetric cells using ZF@F-TiO2anode measured at 1 mV s−1. Peak areas of Zn stripping/plating reactions (c) and corresponding Coulombic efficiency (d) of the prepared Zn anodes in Zn–Zn symmetric cells. There are orthogonal lattice fringes with equal lattice spacing (0.19 nm) inside the nanosheet (Fig. 1i ), corresponding to [1 0 0] and [0 1 0] directions (both belong to <1 0 0> family of directions). Therefore, the normal direction of top surface is [0 0 1] direction perpendicular to both [1 0 0] and [0 1 0] directions [29] . According to the observation of side-view and top-view HRTEM images, it is confirmed that (0 0 1) facet is the highly exposed top surface of F-TiO 2 nanosheet. Another set of orthogonal lattice fringes corresponding to [1 0 1] and [0 1 0] directions (Fig. 1j ) indicates the existence of (1 0 −1) or (−1 0 1) facets (equivalent to (1 0 1) facet because of the tetragonal symmetry) at the edge of nanosheet [30] . Besides, the side surface intersects the top (0 0 1) surface at an obtuse angle (Fig. 1g and Supplementary Fig. 6c ). It can be concluded that the side surface of F-TiO 2 nanosheet is (1 0 1) facet rather than the vertical (1 0 0) facet. The percentage of the exposed (0 0 1) and (1 0 1) facets can be calculated to be 83% and 17%, respectively, by considering the nanosheet as a compressed square frustum. With regard to C-TiO 2 (Supplementary Fig. 7 ), it exhibits a nanoparticle morphology with an average diameter of 20 nm and the irregular lattice fringes indicate its random growth orientation, which leads to more exposure of TiO 2 (1 0 0) facets. The large area of extra TiO 2 (1 0 0) facet is detrimental to prevent the growth of Zn dendrites. Accordingly, it is believed that F-TiO 2 nanosheets with exposed (0 0 1) and (1 0 1) facets can completely shield Zn and restrict the formation of dendrites. Fig. 2: Zn deposition behavior of the prepared anodes. a Schematic illustration of the Zn plating process with different coating layers. b CV curves of Zn–Zn symmetric cells using ZF@F-TiO 2 anode measured at 1 mV s −1 . Peak areas of Zn stripping/plating reactions ( c ) and corresponding Coulombic efficiency ( d ) of the prepared Zn anodes in Zn–Zn symmetric cells. Full size image Electrochemical performance of F-TiO 2 as a protective layer TiO 2 protective layer was introduced on Zn anode by a simple blade coating method and the corresponding XRD pattern (Supplementary Fig. 8 ) demonstrates that the composite Zn anode is successfully synthesized. The Zn plating process on different Zn anodes is illustrated in Fig. 2a . Charges and ions tend to accumulate on the small tips at the surface of commercial Zn foil anodes when there is an impressed voltage. The resulting uneven interfacial electric field and ion concentration can induce preferential Zn growth and eventually lead to the formation of Zn dendrites during the repeated stripping and plating cycles [31] . When using C-TiO 2 as the intermediate layer, Zn tends to grow on the surface of TiO 2 layer with a higher Zn affinity. For comparison, the Zn plating reaction can be well confined under the protective layer and the smooth Zn layer can be deposited on the Zn anode by faceting the TiO 2 to specific orientations with low Zn affinity. The cyclic voltammetry (CV) curves of F-TiO 2 coated Zn foil (ZF@F-TiO 2 ) in Zn–Zn symmetric cells (Fig. 2b ) can almost maintain the identical shapes in comparison with the changed peaks of C-TiO 2 coated Zn foil (ZF@C-TiO 2 ) and Zn foil (ZF) (Supplementary Fig. 9 ), which indicates the superior reversibility of Zn stripping/plating in ZF@F-TiO 2 anode. The peak areas of each redox reaction of CV curves can be obtained by integration operation (Fig. 2c ). The larger peak area of ZF@F-TiO 2 anode reflects the enhanced interfacial activity for Zn deposition [32] . Zn 2+ driven by the electric field and concentration gradient migrate toward the Zn anode and tend to be repulsed by the F-TiO 2 layer at the interface, leading to the Zn 2+ accumulation near the anode surface. The increased Zn 2+ concentration can not only activate more binding sites for Zn deposition but also accelerate the Zn 2+ transfer rate on the surface to alleviate the uneven Zn 2+ distribution, which is beneficial to the ordered interfacial Zn deposition [33] , [34] . Moreover, the highest Coulombic efficiency (reduction/oxidation) of ZF@F-TiO 2 among all the prepared anodes (Fig. 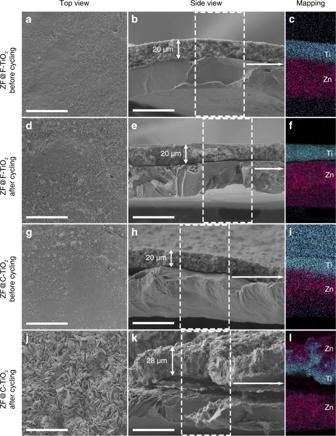Fig. 3: Morphology evolution of the prepared Zn anodes. SEM and the corresponding EDX mapping images ofa–fZF@F-TiO2andg–lZF@C-TiO2before and after 10 cycles in Zn-SS cells. Scale bar: 40 μm. 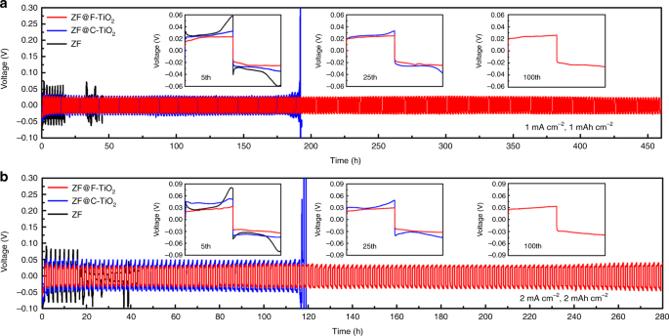Fig. 4: Electrochemical performance of prepared Zn anodes. Cycling performance Zn–Zn symmetric cells ata1 mA cm−2for 1 mAh cm−2andb2 mA cm−2for 2 mAh cm−2. 2d ) is also the evidence of its superior reversibility, which can be ascribed to the more uniform Zn deposition and less formation of “dead Zn”. TiO 2 coated Zn foils exhibit better hydrophilicity than pure Zn foil (Supplementary Fig. 10 ), indicating that electrolyte can penetrate TiO 2 layers to facilitate Zn 2+ transport towards anode surface. The voltage profiles of the first ten cycles of zinc-stainless steel (Zn-SS) cells were recorded, which are shown in Supplementary Fig. 11 . Pure Zn foil fails rapidly within 600 min due to the short circuit caused by the formation of dendrites. And the cycling stability of the cells is significantly improved when Zn foils are coated with the TiO 2 interface layer. Specifically, ZF@F-TiO 2 exhibits longer cycling life than ZF@C-TiO 2 , indicating its better Zn reversibility achieved by the specific exposed facets. Zn anodes were extracted from Zn-SS cells and their digital photographs are shown in Supplementary Fig. 12 . Some unevenly distributed crystals are formed on the surface of ZF and ZF@C-TiO 2 , while ZF@F-TiO 2 can maintain the original structure of F-TiO 2 layer. Scanning electron microscope (SEM) images of these cycled electrodes were also compared with the fresh anodes (Fig. 3 ). The morphologies of ZF@F-TiO 2 and ZF@C-TiO 2 are consistent before cycling. TiO 2 coating layer with a smooth surface and uniform thickness (20 μm) is in close contact with Zn foil. After cycling, there is no obvious change in ZF@F-TiO 2 and its interface is still tightly combined. The well-defined distribution of Ti and Zn in the energy dispersive X-ray (EDX) mapping images (Fig. 3c, f ) also demonstrates the good reversibility during stripping and plating cycles. As shown in Fig. 3j, k , Zn sheets (3μm in length) are observed on the surface of cycled ZF@C-TiO 2 , which is easily turned into Zn dendrites and causes the safety problem. C-TiO 2 layer seems ineffective due to a large amount of Zn transferred from Zn foil and the formation of void space at the interface. The process of Zn transfer to the surface can be seen in the EDX mapping image (Fig. 3l ). Supplementary Fig. 13 exhibits the more disordered surface with the wild growth of Zn dendrites on the cycled pure Zn foil, which is in agreement with the short-circuited Zn-SS cell within 10 cycles. From the different morphologies mentioned above, it is proved that the facet orientation plays an important role in adjusting Zn deposition behavior and TiO 2 protective layer with highly exposed (0 0 1) facet with low Zn affinity can completely confine the Zn deposition in the restricted space. Besides, the TiO 2 layer on the cycled anodes was removed by using methyl-2-pyrrolidinone (NMP) to dissolve polyvinylidene difluoride (PVDF) in the layers. As seen from the SEM images of the Zn surface after cycling (Supplementary Fig. 14 ), Zn deposition in ZF@F-TiO 2 is flat and tends to accumulate parallel to the Zn surface, which also suggests the limited Zn growth by F-TiO 2 protective layer with decreased Zn affinity. Fig. 3: Morphology evolution of the prepared Zn anodes. SEM and the corresponding EDX mapping images of a – f ZF@F-TiO 2 and g – l ZF@C-TiO 2 before and after 10 cycles in Zn-SS cells. Scale bar: 40 μm. Full size image The positive effect of the F-TiO 2 layer on Zn plating behavior was further investigated by testing the cycling stability of Zn anodes in Zn/Zn symmetric cells. As shown in Fig. 4a , ZF@F-TiO 2 can be operated steadily for more than 460 h at 1 mA cm −2 for 1 mAh cm −2 , which is much superior to ZF@C-TiO 2 (190 h) and ZF (20 h). 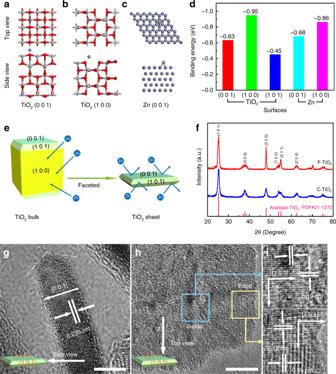When increasing the current density to 2 mA cm −2 and the specific capacity to 2 mAh cm −2 (Fig. 4b ), ZF@F-TiO 2 can still charge and discharge for 280 h in contrast to the quick failure of ZF@C-TiO 2 and ZF with the shorter lifespan of 115 and 15 h, respectively. Besides, ZF@F-TiO 2 exhibits the most stable voltage plateau and the lowest voltage hysteresis, reflecting the enhanced Zn transfer kinetics [35] . Fig. 1: Theoretical simulation and characterization of F-TiO2. Calculations models of Zn absorbed onaTiO2(0 0 1) facet,bTiO2(1 0 0) facet, andcZn (0 0 1) facet.dCalculated binding energies of Zn atom with different facets.eSchematic illustration of the interaction between Zn and anatase TiO2with different exposed facets.fXRD patterns of F-TiO2and C-TiO2.g–jHRTEM images of F-TiO2. Scale bars: 5 nm. The electrochemical performance of ZF@F-TiO 2 is competitive in comparison with several Zn anodes using protective coating materials (Supplementary Table 1 ). The full cells were assembled with the as-prepared Zn anodes and commercial manganese dioxide (MnO 2 ) cathode. The full cell using ZF@C-TiO 2 anode exhibits the lowest polarization voltage and best cycling performance with the capacity retention ratio of 84.1% after 300 cycles (Supplementary Fig. 15 ). The enhanced full cell performance using the F-TiO 2 layer suggests its potential for practical application. Fig. 4: Electrochemical performance of prepared Zn anodes. Cycling performance Zn–Zn symmetric cells at a 1 mA cm −2 for 1 mAh cm −2 and b 2 mA cm −2 for 2 mAh cm −2 . Full size image High-performance Zn anode without external dendrite growth was fabricated by coating TiO 2 with highly exposed (0 0 1) facet on commercial Zn foil. Benefiting from the specific crystal orientation of TiO 2 with abomination to Zn absorption, Zn 2+ transferred by the electric field was enriched on the anode surface. Thus, the increased interfacial Zn 2+ concentration could induce uniform nucleation and the further Zn deposition was guided to grow laterally. The as-prepared Zn anode exhibited superior Zn stripping and plating performance with a long lifespan (460 h at 1 mA cm −2 for 1 mAh cm −2 ). More importantly, the strategy to change the Zn affinity by adjusting the exposure of the facet provides a deep insight into the internal mechanism of metal affinity and can be extended to interfacial modification for other metal anodes. Synthesis of F-TiO 2 Tetrabutyl titanate (10 mL, Aladdin) and hydrofluoric acid (1.2 mL, 40 wt%, Sinopharm) were added into a 50 mL Teflon-lined autoclave and then maintained at 180 °C for 24 h. The precipitates were collected by vacuum filtration then washed by ethanol and dried at 80 °C for 6 h. Fabrication of ZF@F-TiO 2 F-TiO 2 and PVDF were mixed in a weight ratio of 9:1 with NMP as the dispersant. The slurry was pasted onto Zn foil (30 μm) and dried at 80 °C for 24 h under vacuum. For comparison, ZF@C-TiO 2 was also prepared by replacing F-TiO 2 with C-TiO 2 . Characterizations XRD was tested by a Bruker D8 X-ray diffractometer with monochromatized Cu Kα radiation (wavelength = 1.5406 Å). Raman spectra were recorded using a Renishaw inVia spectrometer using an excitation wavelength of 532 nm. Morphologies of the prepared TiO 2 and Zn anodes were characterized by SEM (Nova NanoSEM 230) and TEM (Tecnai G2 F20 S-TWIN). The contact angle was measured by a drop shape analyzer (DSA100). Electrochemical measurements Coin-type cells (CR2025) were assembled for Zn–Zn symmetric cells, Zn-SS half cells and Zn-MnO 2 full cells with glass fiber as separator and 1 M zinc sulfate (ZnSO 4 ) aqueous solution as the electrolyte. Battery performance was evaluated using a Neware battery testing system. CV measurement for Zn–Zn symmetric cells was conducted on a CHI760E electrochemical workstation in the voltage range of −0.1–0.1 V. Zn-SS half cells were cycled with a specific capacity of 1  mAh cm −2 at 1 mA cm −2 for the charging process and a cut-off potential of −0.3 V at 1 mA cm −2 for the discharging process. Full cells were cycled between 1.0 and 2.0 V using commercial MnO 2 (Macklin) as the cathode. In all, 0.1 M manganese sulfate (MnSO 4 ) was added in the ZnSO 4 electrolyte to prevent Mn 2+ dissolution. Computational details The first-principles calculations were conducted using generalized gradient approximation (GGA) and Perdew–Burke–Ernzerhof (PBE) exchange-correlation functional in DMol3 module of Materials Studio (version 8.0) of Accelrys Inc. An all-electron numerical basis set with polarization functions (DNP basis set) and a DFT-D method within the Grimme scheme was employed. The convergence tolerance was set to 1.0 × 10 −5 Ha (1 Ha = 27.21 eV) for energy, 2.0 × 10 −3 Ha Å −1 for maximum force and 5.0 × 10 −3 Å for maximum displacement. Common facets of TiO 2 and Zn were investigated in this simulation, including TiO 2 (0 0 1), TiO 2 (1 0 0), TiO 2 (1 0 1), Zn (0 0 1) and Zn (1 0 0). Each facet was set as a five-layer 3 × 3 supercell with top three-layer atoms releasable. Zn atom was placed in the vertex of the oxygen octahedron of the TiO 2 facet or the tetrahedral vertex of the Zn facet before geometry optimization. Binding energy ( E b ) was calculated by the following equation: 
    E_b = E_total - E_sub-E_Zn
 (2) E total , E sub , and E Zn represent the total energy of the facet combined with Zn atom, the energy of the facet and the energy of Zn atom, respectively.